Selective dispersion of high purity semiconducting single-walled carbon nanotubes with regioregular poly(3-alkylthiophene)s Conjugated polymers, such as polyfluorene and poly(phenylene vinylene), have been used to selectively disperse semiconducting single-walled carbon nanotubes (sc-SWNTs), but these polymers have limited applications in transistors and solar cells. Regioregular poly(3-alkylthiophene)s (rr-P3ATs) are the most widely used materials for organic electronics and have been observed to wrap around SWNTs. However, no sorting of sc-SWNTs has been achieved before. Here we report the application of rr-P3ATs to sort sc-SWNTs. Through rational selection of polymers, solvent and temperature, we achieved highly selective dispersion of sc-SWNTs. Our approach enables direct film preparation after a simple centrifugation step. Using the sorted sc-SWNTs, we fabricate high-performance SWNT network transistors with observed charge-carrier mobility as high as 12 cm 2 V −1 s −1 and on/off ratio of >10 6 . Our method offers a facile and a scalable route for separating sc-SWNTs and fabrication of electronic devices. Single-walled carbon nanotubes (SWNTs) have a wide range of extraordinary mechanical, chemical and electronic properties [1] , making them ideal candidates for various applications, such as composites [2] , energy storage [3] , biological and chemical sensors [4] , [5] , [6] , [7] , flexible electronics [8] , [9] and transparent electrodes [10] , [11] . In particular, the high charge-carrier mobility of semiconducting (sc-) SWNTs together with the ability for solution processing hold a great promise for high-performance low-cost transistor applications. Despite their immense potential, separating sc-SWNTs from metallic (met-) SWNTs from an as-synthesized mixture in high yields remains a challenge [12] , [13] , [14] , [15] , [16] , [17] , [18] , [19] , [20] , [21] . Great progress has been made to develop advanced selective growth methods [22] , [23] , [24] , [25] , [26] , [27] . However, further improvements in both afforded yields and subsequently scaling-up processes are still needed. Postgrowth separation is an alternative technique that resulted in the enrichment of sc-SWNTs [13] , [14] , [17] , [18] , [20] , [21] , [28] , [29] . Despite their promises, each method still has its own limitations in scaling up and/or requires the tedious process of removing the insulating surfactants or polymers. Conjugated polymers, with extensive π-conjugated structures, have been reported to interact strongly with SWNTs [18] , [30] , [31] , [32] , [33] , [34] . Although polymers, such as poly(9,9-dialkyl-fluorene) derivatives, were found to disperse sc-SWNTs [18] , making high-performance devices is challenging due to difficulty in removing these insulating polymers. Recently, polymers such as poly(m-pheneylene vinylene)s were shown to selectively disperse certain chiralities of SWNTs, and it was reported that the ability for the polymer to adapt a helical conformation is critical for effective SWNT dispersion and/or sorting [35] . Among the semiconducting polymers, regioregular poly(3-alkylthiophene)s (rr-P3ATs, Fig. 1a ) possess both high charge-carrier mobility in thin-film transistors (TFTs) and excellent power conversion efficiency in heterojunction solar cells [36] , [37] . rr-P3ATs are also known to self-organize into highly ordered structures in both thin film and on SWNTs [36] . Polythiophenes have previously been used to increase the dispersion concentration of SWNTs [11] , [38] , [39] , but their application towards selective dispersion of SWNTs has not been reported. 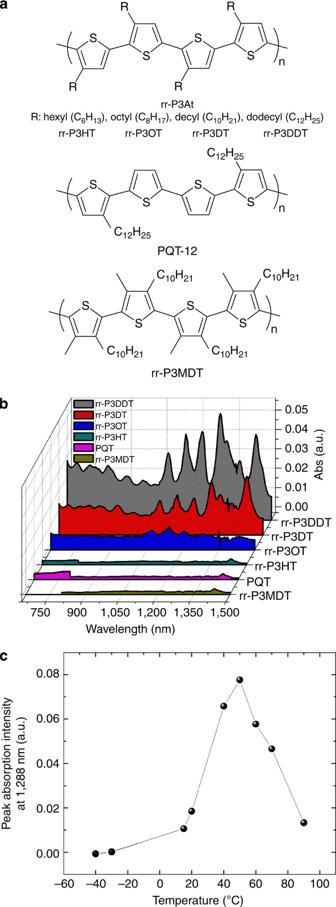Figure 1: Chemical structures and absoprtion data of the various studied polymers. (a) Chemical structures of the various polythiophenes investigated. (b) Absorption spectra of the supernatants collected after centrifugation of the polythiophenes–SWNT suspensions. (c) Absorption intensities at 1288 nm from the supernatants of rr-P3DDT/SWNT, dispersed from −40 to 90 °C. Figure 1: Chemical structures and absoprtion data of the various studied polymers. ( a ) Chemical structures of the various polythiophenes investigated. ( b ) Absorption spectra of the supernatants collected after centrifugation of the polythiophenes–SWNT suspensions. ( c ) Absorption intensities at 1288 nm from the supernatants of rr-P3DDT/SWNT, dispersed from −40 to 90 °C. Full size image Here we describe the selective dispersion of sc-SWNTs using the regioregular poly(3-dodecylthiophene) (rr-P3DDT). Through rational selection of polymers, solvent and temperature, we achieved highly selective dispersion of sc-SWNTs. Our approach enables direct film preparation after a simple centrifugation step. The sorted sc-SWNTs resulted in high-performance SWNT network transistors with an observed charge-carrier mobility as high as 12 cm 2 V −1 s −1 and on/off ratio of >10 6 . Dispersion with various polythiophene derivatives Commercially available High-Pressure CO (HiPCO) SWNTs were first dispersed using several polythiophene derivatives ( Fig. 1a , molecular weight and polydispersity values are listed in Supplementary Table S1 ) in toluene at temperatures measured in the dispersions ranging from −40 to 90 °C during sonication with an ultrasonicator for ~30 min. A typical experimental apparatus is depicted in Supplementary Figure S1 . After centrifugation, ultraviolet/Visible/Near Infrared (UV/Vis/NIR) spectroscopy was taken on the supernatants to measure the relative amounts of dispersed SWNTs in various polythiophene derivatives ( Fig. 1b ). The absorption of the polythiophene is confined to the visible region, while the absorption from the SWNTs extends into the NIR region. We observed that the rr-P3DDT solution (without SWNTs, concentration of 0.4 mg ml −1 ) showed only a single absorption peak at ~450 nm ( Supplementary Fig. S2 ). On the other hand, we observed absorption peaks at ~450 nm along with vibronic peaks for rr-P3DDT at both 553 and 602 nm for the SWNT/rr-P3DDT solution and the rr-P3DDT film. The additional vibronic peaks observed suggest that the polymer is now strongly bound to the SWNTs (in the case of the SWNT/rr-P3DDT solution) or the substrate (in the case of rr-P3DDT film), and the motion of the polymer backbones are subsequently restricted [40] . As shown in Figure 1b , we observed the strongest SWNT peak intensity at NIR region for rr-P3DDT supernatant, indicating that a higher percentage of SWNTs was dispersed with rr-P3DDT (contains –C 12 H 25 side chains), as compared with the other polythiophene derivatives. For other rr-P3AT derivatives with smaller side chains, the SWNT dispersions were significantly lower. In particular, rr-P3OT (contains –C 8 H 17 side chains) and rr-P3HT (contains –C 6 H 13 side chains) barely showed any SWNTs dispersion under the same experimental conditions ( Fig. 1b ). Interestingly, no SWNT was dispersed (as no absorption peaks were observed) with the polymers regioregular poly(3-methyl-4-decyl-thiophene-2,5-diyl) (rr-P3MDT), poly(3,3′′′-didodecyl-quarter-thiophene) (PQT-12) and regiorandom P3DDT. Collectively, these results indicate that parameters, such as alkyl chain length, configuration, and density of side chains are all highly important in determining the polymer interaction with the SWNTs. These interactions are important as we found (discussed later) that it is necessary for the formation of an ordered supramolecular structure consisting of the polymer 'wrapped' around the SWNT in order for effective dispersion and sorting. Another important parameter, besides the polymer structure, is the temperature used during sonication. As shown in Figure 1c , the absorption intensity for rr-P3DDT is the highest at a dispersion solution temperature of 50 °C (studied from −40 to 90 °C). This temperature coincides with the side chain melting temperature for the rr-P3DDT [41] , which is measured using differential scanning calorimetry (DSC; Supplementary Fig. S3 ). Similar side chain melting transition was measured with rr-P3DT (C 10 H 21 ), and this polymer was observed to enable dispersion for a small amount of SWNTs. As for polymers rr-P3OT (C 8 H 17 ) and rr-P3HT (C 6 H 13 ), no side chain melting transition was observed using DSC. Interestingly, these two polymers were unable to disperse many SWNTs. Spectroscopic characterization of sorted SWNTs To identify the electric types of SWNTs dispersed with rr-P3DDT in toluene at 50 °C, we performed resonant Raman scattering (RRS) measurements ( Fig. 2 ; Supplementary Figs S4, S5 ) using three excitation energies, namely, at 2.33 eV (532 nm), 1.96 eV (633 nm) and 1.58 eV (785 nm). We assign both the chiralities and electric types (that is, met or sc) of the SWNTs using the revised Kataura plot ( Supplementary Tables S2-S6 ) [14] . The 2.33 eV excitation line is mainly in resonance with met-SWNTs within the range of radial breathing mode peaks from 180 to 280 cm −1 . The supernatants measured indicate that all the peaks in the metallic region, which were originally present in the unsorted tubes, have all disappeared before and after polymer burn off ( Fig. 2a ; Supplementary Fig. S5 ). This indicates that the met-SWNTs resonant with 2.33 eV excitation have been completely removed and only sc-SWNTs remained. 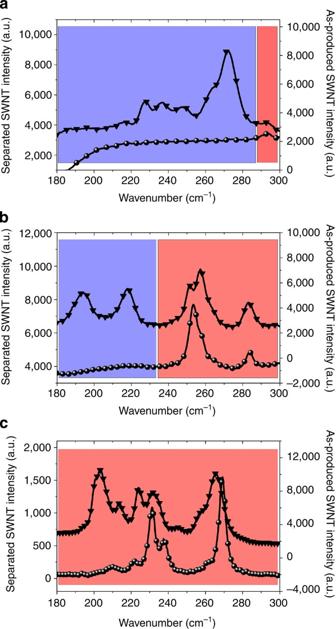Figure 2: Radial breathing mode (RBM) regions of resonant Raman scattering spectra at three excitation energies. (a) 2.33 eV (532 nm) is mainly resonant with met-SWNTs (blue shaded) in the range of 180–285 cm−1, (b) 1.96 eV (633 nm) is resonant with met-SWNTs and sc-SWNTs (red shaded) in ~1:1 ratio, (c) 1.58 eV (785 nm) is resonant with sc-SWNTs. The peak intensities of the SWNTs with the diameter distribution between 0.88 and 1 nm were enhanced after sorting. In each spectrum, the upper RBM profile (black triangle) and the lower profile (black sphere) represent before and after sorting, respectively. The assignments of peaks can be found inSupplementary Tables S3-S5. Figure 2: Radial breathing mode (RBM) regions of resonant Raman scattering spectra at three excitation energies. ( a ) 2.33 eV (532 nm) is mainly resonant with met-SWNTs (blue shaded) in the range of 180–285 cm −1 , ( b ) 1.96 eV (633 nm) is resonant with met-SWNTs and sc-SWNTs (red shaded) in ~1:1 ratio, ( c ) 1.58 eV (785 nm) is resonant with sc-SWNTs. The peak intensities of the SWNTs with the diameter distribution between 0.88 and 1 nm were enhanced after sorting. In each spectrum, the upper RBM profile (black triangle) and the lower profile (black sphere) represent before and after sorting, respectively. The assignments of peaks can be found in Supplementary Tables S3-S5 . Full size image Subsequently, with excitation energy of 1.96 eV, resonance for both met- and sc-SWNTs (in ~1:1 ratio) was observed for the unsorted SWNTs ( Fig. 2b ; Supplementary Fig. S5 ). After sorting, the spectrum again indicates that the met-SWNTs (both (9,9) and (12,3) types) were removed from the supernatant and only the sc-SWNTs remained. Finally, only sc-SWNTs were observed using excitation energy of 1.58 eV ( Fig. 2c ; Supplementary Fig. S5 ). In addition, we observed that for the sorted sc-SWNTs, the fraction with the larger diameter SWNTs (~1.1 nm) was reduced, while only the smaller diameter sc-SWNTs (0.88–1 nm) remained in the supernatant. Much sharper radial breathing mode peaks for the sorted sc-SWNTs were also observed, which indicates that the nanotubes are primarily unbundled (or unaggregated). Upon further examination with atomic force microscopy (AFM), the obtained images indeed indicate unbundled nanotubes with an average height and length of 1.6 nm and 1 μm, respectively ( Supplementary Fig. S6 ). We note that as the average height of each of the unbundled nanotube is ~0.8 to 1.0 nm. Our slightly larger observed height for our nanotubes is attributed to the polymers wrapping around the SWNTs. UV/Vis/NIR spectrum of sorted SWNTs after polymer burn off offers additional support for dispersion of sc-SWNTs. As shown in Supplementary Figure S7 , the peaks originally present in the M11 region all disappeared for sorted SWNTs. The estimated yield for sorted sc-SWNT was ~19% in weight. Hence, no significant enrichment of metallic tubes was observed for the sediment layer. However, the sorting yield can potentially be improved by increasing sonication power, increasing polymer to carbon nanotube (CNT) ratio and using other solvents. As Raman spectroscopy can only identify SWNTs that are in resonance with the laser excitation wavelengths, we have used photoluminescence excitation/emission (PLE; Fig. 3 ; Supplementary Figs S8, S9 ) to further determine the different chiralities of SWNTs dispersed with rr-P3DDT, and compared it with SWNTs dispersed with sodium dodecyl sulphate (SDS; which has been previously reported to not show any selective sorting) [42] . 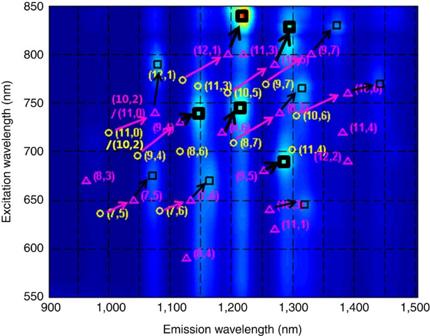Figure 3: Photoluminescence excitation/emission (PLE) data map for SWNT dispersed with rr-P3DDT in toluene at 50 °C. Yellow circles indicate 'air-suspended SWNT,' purple triangles indicate 'SWNT dispersed with SDS in water,' black squares indicate 'SWNT dispersed with rr-P3DDT in toluene' and bold black squares indicate 'SWNT dispersed in rr-P3DDT in relatively higher concentrations.' As the PLE data indicate in Figure 3 , the dominant SWNTs dispersed with rr-P3DDT were (12,1), (10,5), (8,6), (9,4) and (9,5). On the other hand, SDS/water dispersed a wide variety of SWNTs ( Supplementary Figs S8, S9 ). Interestingly, we observed that there was a systematic redshift of both the excitation (~25 to 30 meV) and emission peaks (~50 to 60 meV) for SWNTs dispersed with rr-PDDT in toluene, compared with those dispersed in SDS/water ( Fig. 3 ; Supplementary Fig. S8 ). This redshift has previously been reported and was attributed to dielectric screening [40] , which results from the interaction of the polymer with SWNTs. Figure 3: Photoluminescence excitation/emission (PLE) data map for SWNT dispersed with rr-P3DDT in toluene at 50 °C. Yellow circles indicate 'air-suspended SWNT,' purple triangles indicate 'SWNT dispersed with SDS in water,' black squares indicate 'SWNT dispersed with rr-P3DDT in toluene' and bold black squares indicate 'SWNT dispersed in rr-P3DDT in relatively higher concentrations.' 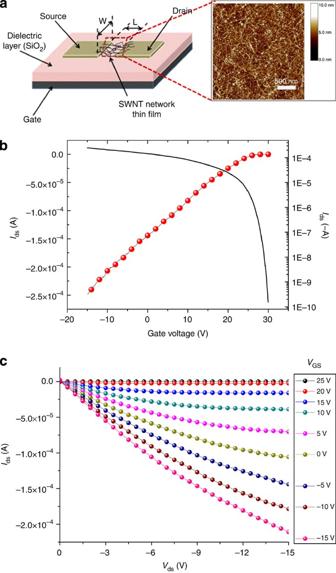Figure 4: Thin-film transistor schematics and measurements. (a) Schematic of a SWNT thin-film transistor. Pt/Ti electrodes for source and drain were patterned with 10 μm of channel length on a heavily n-doped Si substrate as the gate and a 300 nm SiO2as the dielectric layer. The SiO2surface was modified by an amine-terminated self-assembled monolayer. The SWNT film was deposited by soaking the substrates in the polymer/sc-SWNT dispersion, and (insert) the AFM image of the SWNT network deposited in a thin-film transistor is measured in the channel region. (b) A current–voltage characteristic for a transistor with a mobility ~12 cm2V−1s−1and an on/off ratio ~106. The drain-source voltage used is −15 V. (c) The output curve of the transistor. Full size image Thin-film transistor characterization of sorted SWNTs To further confirm that selective sorting of sc-SWNTs was achieved, we fabricated SWNT network TFTs on a highly doped Si substrate as the gate electrode and SiO 2 (300 nm) as the dielectric layer, as depicted in Figure 4a . The average SWNT length is 1.0±0.1 μm, as measured from 141 randomly selected SWNTs using scanning electron microscopy ( Supplementary Fig. S6 ). In all these devices, the SWNTs were observed to be fully percolating within the channel with a channel length of 1.5 μm, at a coverage of >50 SWNTs per μm 2 in a single layer and a thickness of ~2.3 nm as measured by AFM. Figure 4: Thin-film transistor schematics and measurements. ( a ) Schematic of a SWNT thin-film transistor. Pt/Ti electrodes for source and drain were patterned with 10 μm of channel length on a heavily n-doped Si substrate as the gate and a 300 nm SiO 2 as the dielectric layer. The SiO 2 surface was modified by an amine-terminated self-assembled monolayer. The SWNT film was deposited by soaking the substrates in the polymer/sc-SWNT dispersion, and (insert) the AFM image of the SWNT network deposited in a thin-film transistor is measured in the channel region. ( b ) A current–voltage characteristic for a transistor with a mobility ~12 cm 2 V −1 s −1 and an on/off ratio ~10 6 . The drain-source voltage used is −15 V. ( c ) The output curve of the transistor. Full size image Among 122 randomly chosen devices, no device shorting was observed and an average on/off ratio of ~10 4 was recorded ( Supplementary Fig. S10 ). In addition, hole mobility as high as 12 cm 2 V −1 s −1 with an on/off current ratio of ~10 6 were obtained without any 'burn-off' or posttreatment ( Fig. 4b,c ). We also measured 12 devices at random. The average for the on/off ratio was 3×10 6 and the average mobility was 8.5 cm 2 V −1 s −1 . The observed positive threshold voltage is attributed to a combination of oxygen and water doping in ambient air, and doping by the polymer rr-PDDT, in which both doping processes have been previously reported for CNT-based transistors [43] . Device operation in an inert atmosphere will significantly reduce this phenomenon, but it may not be a practical approach for certain applications. Polymer or atomic layer deposition passivation can be used to reduce this effect [44] , [45] . Threshold voltage can also be controlled by dielectric surface modification with self-assembled monolayers with electrical dipoles [46] , polarization effects [47] , electrostatic doping by high dielectric constant dielectrics, or by using different metal contacts [48] , [49] . The observed values of our fabricated devices, namely for both mobility and on/off ratio, are very good for solution-sorted sc-SWNT networks [20] , [50] , [51] . We anticipate that higher mobility could be attained on further optimization of the SWNT network morphologies, as well as the various dispersion conditions. Also, a previous report has indicated that addition of a small percentage of met-SWNTs will also enhance the mobility without compromising the on/off ratio [50] . Finally, we fabricated single tube devices with 200–300 nm channel length; however, we did not observe any metallic characteristics for the ~80 randomly selected tubes ( Supplementary Fig. S11 ). This again supports the conclusion that the supernatant is highly enriched with sc-SWNTs. Taken together, our collected spectroscopy and electrical data both strongly support the conclusion that rr-P3DDT is capable of highly selective dispersion of sc-SWNTs under a set of prescribed parameters. We note that toluene is the preferred solvent for the sorting process because the solubility of SWNTs in toluene is poor. Addition of polymers can hence result in their subsequent dispersion. We also note that chlorinated solvents can disperse SWNTs even without addition of polymer, thus they are not effective for usage in selective sorting. The interaction between our added polymer and SWNTs is important in determining the amount and the type of SWNTs dispersed. As already mentioned, the chain length of the rr-P3ATs has a direct impact on the dispersion of SWNTs. We suspect that on wrapping of the side chain around the SWNT, a 'polymer shell' was rendered around the SWNT. The correlation between the optimal dispersion temperature and the side chain melting transition temperature, as observed by DSC, suggests that it is important for the side chains to maintain a certain degree of flexibility to assume optimized supramolecular assembly, thus encapsulating the dispersed SWNT. At a lower temperature, the side chains may have limited movement to either break apart from the existing polymer aggregation or to form the supramolecular structure around the SWNTs; while at higher temperatures, their higher degree of freedom to move around may prevent them from forming an ordered structure. Coupled with our experimental observations that no SWNTs were dispersed by short side-chain-containing polymers, such as rr-P3OT and rr-P3HT, a 'polymer shell' with appropriate diameter is thus important for proper dispersion of the SWNTs. The observation of the optimal dispersion temperature at 50 °C (which coincidentally is also the side-chain melting temperature) may arise due to the competition between several competing thermodynamic and kinetic effects. At high temperatures, the side-chain fluctuations may prohibit the polymer from adopting wrapped configurations, thus disrupting the supramolecular assembly that would shield favourable SWNT–SWNT interactions. In addition, the entropic benefit for the polymer backbone to explore a multitude of conformations would supersede the propensity for the wrapping of polymer around the SWNT. 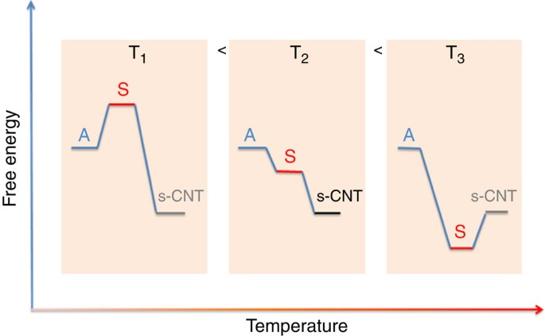Figure 5: Schematic representation of the relative free energies. Free energies (F) of solid polymer aggregate (A), the polymer in solution (S), and the CNT+wrapped polymer in solution (s-CNT) as a function of temperature. The optimal dispersion temperature (T) must satisfy the condition: FA>Fs>Fs−CNT(centre panel). This state of high temperature is schematically depicted in Figure 5 as T 3 . Here, the free energy of the polymer in solution (F s ) is less than the free energy of the CNT+wrapped polymer in solution (F s−CNT ); in other words, it is thermodynamically more stable for the polymer to be in solution than wrapped around the CNT. Figure 5: Schematic representation of the relative free energies. Free energies (F) of solid polymer aggregate (A), the polymer in solution (S), and the CNT+wrapped polymer in solution (s-CNT) as a function of temperature. The optimal dispersion temperature (T) must satisfy the condition: F A >F s >F s−CNT (centre panel). Full size image On the other hand, if the temperature is too low (T 1 ), the free energy of the solid polymer aggregate (F A ) is less than F S ; thus the polymer aggregate is more stable than the polymer in solution. Even if the free energy of the CNT with a wrapped polymer shell (F s−CNT ) is lower than that of the solid polymer aggregate, the wrapping process does not occur because the barrier (F s −F A ) is too high. Polymer wrapping may also be kinetically limited at low temperatures due to the lack of backbone freedom during the wrapping process. This lack of conformational freedom may limit the polymer backbones from eliminating loops, entanglements and other defects around the SWNT, resulting in exposed binding regions that lead to favourable polymer–polymer interactions and consequent aggregation. If the dispersion temperature is such that F A >F s >F s−CNT (T 2 ), then a polymer shell may be formed around the CNT, provided the geometrical criteria discussed in the manuscript are satisfied. In summary, we conclude that the optimal temperature for the CNT dispersion is related to the optimal temperature for the polymer to wrap around the CNT, which requires thermodynamic stability and moderate geometrical freedom of the polymer backbone and side chains. We speculate from our data ( Supplementary Fig. S3 ; Fig. 1c ) that at the side-chain melting temperature, such thermodynamic and kinetic conditions are satisfied. However, although the optimal dispersion temperature and the side-chain melting temperature are suggestively related from our experimental data, their exact correlation is yet to be fully elucidated. It is thus the subject of future work. We also observed that polymer PQT-12, even though the length of its side chain is the same as rr-P3DDT, did not yield any dispersion of SWNTs. This may be due to the fact that PQT-12 has a fewer number of side chains, as only the first and fourth thiophene ring in each repeating monomer contains a side chain (as opposed to rr-P3DDT, in which all the thiophene rings contain a side chain; Fig. 1a for chemical structures). Hence, the number of side chains for PQT-12 may be insufficient to yield a strong enough interaction with SWNT to enable a highly ordered supramolecular structure. We note that the proposed supramolecular structure for polythiophene may not be readily formed in solution in the absence of SWNTs. Similar to other molecules, such as Flavin [19] , where supramolecular assembly is induced by SWNTs, it is thus reasonable to assume that SWNTs may serve as a 'framework' to promote polymer–SWNT supramolecular conformation. 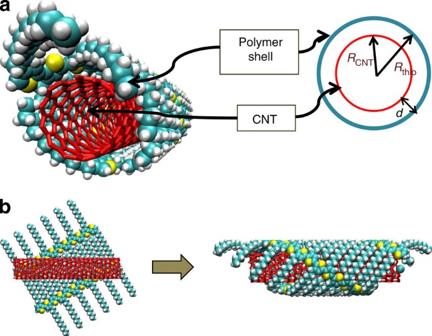Figure 6: Geometric models of the polymer–SWNT supramolecular structure. (a) Schematics of a cross-sectional geometrical view of the polymer–SWNT supramolecular structure, in which the red double-headed arrow 'd' represents the gap between the radii of SWNT and the polymer tubular structure, and (b) based on our modelling studies, the interdigitation of the polymer's side chain causes the formation of a double-stranded polymer, which in turns proceed to wrap around the SWNT. To explain our hypothesis of the 'polymer shell', we devised a geometrical model as shown in Figure 6 . This model is intended to address the likely geometry of the wrapped polymer configuration around a smooth cylinder with a fixed diameter. Our geometrical model is different from the one introduced by Coleman and Ferreira [52] , which identifies energetically favourable coiling angles based on geometric constraints. In our case, we made assumptions on the possible polymer wrapping structures, either single and double strand with side chains interdigitated, based on the previous ultra-high-vacuum scanning tunnelling microscopy results by Giulianini et al [33] . The side-chain interdigitation is also supported by our own observation that the maximum dispersion concentration took place at around the same temperature for side-chain melting, indicating that the side-chain interaction places an important role in the polymer interaction with the SWNTs. This model does not consider the molecular interactions between the polymer and the SWNT. Therefore, it does not explain why the sorting is selective for semiconducting versus metallic SWNTs. Figure 6: Geometric models of the polymer–SWNT supramolecular structure. ( a ) Schematics of a cross-sectional geometrical view of the polymer–SWNT supramolecular structure, in which the red double-headed arrow ' d ' represents the gap between the radii of SWNT and the polymer tubular structure, and ( b ) based on our modelling studies, the interdigitation of the polymer's side chain causes the formation of a double-stranded polymer, which in turns proceed to wrap around the SWNT. Full size image The geometrical model was devised based on the following: First, based on previous experimental observations, we assume that the polymer is able to wrap around a single SWNT [33] , [53] . Giulianini et al [33] reported a detailed experimental evidence of the regioregular poly(3-hexylthiophene) helical wrapping on CNTs by atomically resolved ultra-high-vacuum scanning tunnelling microscopy images. Second, we assume a polymer–SWNT distance ( d ) equal to 3.4 Å, as estimated from ab-initio calculations of the equilibrium distance between graphene and butane (widely used as a model for alkyl side chains). For a given side-chain length (for example, dodecyl), we determined the geometrical conditions, in terms of side-chain length and CNT radius ( R CNT ), leading to a perfectly wrapped polymer on the SWNT. Hence, the radius of the polymer shell determines the diameter (and chirality) of the SWNT that can be encapsulated by the polymer (see detailed explanations about the calculation in Supplementary Tables S7-S9 ). From the above geometrical model, a supramolecular structure consisted of two strands of polymers wrapped around the SWNT with their side chains interdigitated predicted all the experimentally observed sorted sc-SWNTs ( Fig. 6 ; Supplementary Tables S7-S9 ), consistent with UV/Vis/NIR, PLE and Raman measurements. We note that through simultaneous molecular dynamics simulations of polymer–CNT interactions different polymer conformations are possible (including disordered configurations) [54] . However, our geometrical model has predicted a highly ordered supramolecular conformation that is very similar to the conformations obtained from previous AFM and STM experiments [33] , [55] . In addition, the geometrical model is unable to generate any ordered conformations stemming from SWNTs and regiorandom-P3DDT and rr-P3MDT. Interestingly, we were indeed unable to disperse any SWNT with neither regiorandom-P3DDT nor rr-P3MDT (additional methyl groups at the 3-positions, Supplementary Fig. S12 ). We attribute this to the distorted conformations of both polymers' backbones preventing them from forming highly ordered supramolecular conformation around the SWNTs. The geometrical model, however, is insufficient to account for why only sc-SWNTs are dispersed. Although it is possible that the side chains of the polymer may have a role in sorting sc-SWNTs, our ab-initio total energy calculations did not show appreciable energy difference between binding energies of side chains interacting with either the sc- or met-SWNTs. Instead, previous literatures have indicated that the exclusion of met-SWNT may be in fact due to the charge transfer between the met-SWNT and the polymer. From both previous theoretical and experimental studies of met-SWNT [56] , [57] , a charge transfer was observed at the met-SWNT/polymer interface, while there is negligible charge transfer with sc-SWNT. We hypothesize that the charge transfer leads to an interface dipole that may favour a planar π-stacking between the polymer and SWNT, rather than a helical wrapping conformation. Therefore, charge transfer may prevent the supramolecular structure formation needed for dispersing the met-SWNTs. The accurate determination of the difference in charge transfer between sc- and met-SWNTs would require calculations at several levels of theory for the composite system involving the SWNTs and the entire polymer; thus, it would require an extensive amount of computing time to prove this hypothesis, which is a subject for future investigation. In summary, we report a convenient and effective approach to achieve highly selective dispersion of sc-SWNTs with commercially available HiPCO SWNTs, using rr-P3DDT at a dispersing temperature of ~50 °C in toluene. Our geometrical model suggests that selective dispersion is achieved due to the formation of a supramolecular structure, formed via the interdigitation of side chains ( Fig. 6 ) wrapping around the SWNTs. The wrapping process induces the formation of a 'polymer shell' such that the shell diameter matches well with the selected SWNTs. Our studies also indicate that side-chain length, conformation and density of side chains are all important parameters that govern the ability for conjugated polymers to form desired supramolecular structures with certain SWNTs to achieve selective dispersion. Specifically, side chains with more than ten carbon atoms may be an important design rule: the side-chain melting transition and optimal side-chain length will allow formation of an ordered supramolecular 'polymer shell' structure. Therefore, optimal temperature for selective dispersion, another crucial parameter previously ignored, is needed. Our sorted sc-SWNTs are subsequently used to prepare transistors that demonstrate high mobility and high on/off ratio values, without the need for additional processes such as polymer removal or burn-off. In addition, the polymer/SWNT supramolecular structure may be potentially interesting for templated growth of other materials and devices. Our described approach in using polythiophene derivatives, one of the most promising materials in organic electronics, demonstrates efficient sc-SWNT sorting via the formation of polythiophene/sc-SWNT composites. This rapid sc-SWNT sorting process should allow future electronic device applications. Materials The rr-P3ATs were purchased from Sigma-Aldrich, and PQT-12 and rr-P3MDT were purchased from American Dye Source. The molecular weight of each polymer was measured by using gel permeation chromatography and summarized in Supplementary Table S1 . Purified HiPCO SWNT was purchased from Unidym and was used as received. Polymer-assisted dispersion of carbon nanotubes The HiPCO SWNT (5 mg) and the polymer (10 mg) were suspended in toluene (25 ml). This suspension was kept in a temperature-controlled cooling bath and sonicated (Ultrasonic Processor, 750 W; Cole Parmer) for 30 min at an amplitude level of 70% ( Supplementary Fig. S1 ). The solution was subsequently centrifuged (Sorvall RC5C-plus) for 150 min at 42,000 g to remove SWNT bundles and insoluble materials. The supernatant was collected for further analysis. For comparison, an SDS-assisted SWNT dispersion was prepared (2 mg SWNT: 200 mg SDS from J.T. Baker) in water. Sonication was carried out for 30 min in an ultrasonic bath at room temperature. The suspension was centrifuged at 100,000 g for 2 h. To determine the yield for sorted sc-SWNTs, a bulky paper of sorted sc-SWNT was prepared by filtering the supernatant through a filter paper. The bulky paper was rinsed extensively with hot toluene until the filtrate was colourless to remove any residue polymer. It was dried under vacuum and the weight was measured to give a 19% yield of sc-SWNTs (weight ratio of sc-SWNT and the initial unsorted SWNT). This is a conservative estimate as some CNTs were rinsed away during the hot toluene rinse. UV/VIS/NIR absorption spectroscopy The ultraviolet/Vis/NIR measurements of the SWNT dispersions were carried out in 1-mm path-length quartz cells by using a Cary 6000i spectrophotometer (Varian) with toluene as the background. The absorption spectra showed distinct peaks of dispersed individual SWNTs in the range of 300–1,500 nm. Photoluminescence excitation/emission spectroscopy The PLE measurements were performed by using the Nanolog spectrofluorometer for nanomaterials (Horiba Jobin Yvon). A 450-W broadband cw Xenon lamp and a monochrometer supplied the excitation light in the range of 550–845 nm with 5 nm steps. This light illuminated the sample through a quartz fluorescence cell. Photoluminescence was detected at 90° angle with an IGA-3000 liquid nitrogen-cooled InGaAs photodiode array. Resonant Raman scattering The RRS (Model: LabRam Aramis from Horiba Jobin Yvon) was carried out at 2.33 eV (532 nm), 1.96 eV (633 nm) and 1.58 eV (785 nm) excitation at ×100 magnification and 1-μm spot size, and 1,200 grating. Excitation power was 3 mW for the 2.33 eV line, 5 mW for the 1.96 eV line and 25 mW for the 1.58 eV line. The peak positions were calibrated with the Si line at 521 cm −1 . Thin-film transistor fabrication and characterization For 1.5-μm channel length devices, Ti (10 nm)/Pt (25 nm) top-contact electrodes were photolithographically patterned on SWNT films. The dielectric layer was a 300-nm SiO 2 layer on a heavily n-doped Si substrate as the bottom gate. The SiO 2 surface was modified with 3-aminopropyltrimethoxysilane by soaking the substrate into a solution of 1% 3-aminopropyltrimethoxysilane (Gelest) in anhydrous toluene at room temperature for 1 h. Subsequently, the substrate was rinsed several times with anhydrous toluene and annealed in vacuum over for 30 min at 100 °C. The sorted sc-SWNTs in toluene were deposited onto the substrate by soaking in supernatant (1:100 dilution with toluene for 12 h). Before electrical measurements, the sample was annealed at 110 °C in vacuum to remove toluene. A Keithley 4,200 SC semiconductor analyzer was used to measure the electrical properties of the devices. Ab-initio calculations The first principle calculation discussed in the manuscript has been carried out using density functional theory, in the local density approximation (LDA). We chose the LDA as it yields the results closest to those of accurate quantum monte carlo calculations for graphitic-like systems. Geometrical modelling This model is intended to address the likely geometry of the wrapped polymer configuration around a smooth cylinder with a fixed diameter. This model does not consider the molecular interactions between the polymer and the SWNT. On the basis of the previous experimental observations that regioregular poly(3-hexylthiophene) is able to wrap around a single SWNT [33] , [53] , we assume that SWNTs are selected in a geometrical configuration where the polymer perfectly wraps around the tube, and we compute the mismatch between the tube and the wrapped polymer: where where p and q are the (integer) indices of the polymer shell ( Fig. 6 ). The parameter p denotes the multiplicity of the polymer helix (single stranded: p =1, double stranded: p =2, and so on). The parameter q denotes the periodicity of the helix ( q pairs of thiophene rings per turn). where we chose d CC =1.42 Å and m and n are the indices of the CNT. The interchain spacing a is assumed to depend on the side-chain length in the following way: where N s is the length of side chains (number of C atoms) and the parameters 2.38 and 10.95 (related to side-chain spacing and length) have been estimated from data in the literature (both theory and experiment). The parameter b is the period of the polymer backbone (length of two thiophene units) b = 14.56 (a.u.). The value of b has been determined by carrying our density functional theory calculations within the LDA calculation of a p =0, q =6 polymer shell. The geometry of the polymer shell was relaxed. The distance d is taken to be d =6.4 (a.u.). This value has been determined by computing an alkane–graphene distance within LDA, and by taking this as representative of the distance between side chains and the CNT. The supplementary Tables S6-S9 give: m , n , p , q , N s , R cnt , R thio , Θ (wrapping angle of the polymer), and mismatch (Δ R ). Only combinations with mismatch smaller than 0.3 are shown. We distinguish between semiconducting (SC) tubes selected by the model, SC tubes eliminated by the model and metallic (M) tubes eliminated by the model. The semiconducting tubes selected by the model are summarized in Supplementary Table S7 . Metallic tubes are all eliminated in the experiment. However, five (out of seven) metallic tubes have a mismatch smaller than 0.21 and are therefore selected by the model. How to cite this article: Lee, H. W. et al . Selective dispersion of high purity semiconducting single-walled carbon nanotubes with regioregular poly(3-alkylthiophene)s. Nat. Commun. 2:541 doi: 10.1038/ncomms1545 (2011).